Determination of energy level alignment at metal/molecule interfaces by in-device electrical spectroscopy The energetics of metal/molecular semiconductor interfaces plays a fundamental role in organic electronics, determining the performance of very diverse devices. So far, information about the energy level alignment has been most commonly gained by spectroscopy techniques that typically require experimental conditions far from the real device operation. Here we demonstrate that a simple three-terminal device allows the acquisition of spectroscopic information about the metal/molecule energy alignment in real operative condition. As a proof of principle, we employ the proposed device to measure the energy barrier height between different clean metals and C 60 molecules and we recover typical results from photoemission spectroscopy. The device is designed to inject a hot electron current directly into the molecular level devoted to charge transport, disentangling the contributions of both the interface and the bulk to the device total resistance, with important implications for spintronics and low-temperature physics. The energetics of metal/molecule interfaces has been the subject of intensive study over the past two decades [1] , [2] . Significant energy barriers build up between the metal Fermi energy and the molecular levels devoted to charge transport, limiting the charge injection from the metals to the molecular semiconductors. These energy barriers have a deep impact on the performances of devices, determining the operation voltage in organic light emitting diodes [3] , the threshold voltage of field-effect transistors [4] and the open circuit voltages in photovoltaic devices [5] . Therefore, an accurate knowledge of the energetics is necessary for the engineering of metal–molecule interfaces and the consequent optimization of the device performances. Different approaches have been applied to the study of metal/molecule interfaces, such as electron photoemission spectroscopy [1] , [2] and Kelvin probe measurements [6] . In such experiments the energy level alignment is typically extracted by monitoring the change in the work function when thin molecular layers are evaporated on to the surface of a metal. Therefore, it is not possible to monitor directly how the measured energy level alignment reflects on to the electrical charge injection. In this sense, it is of major interest to gain the same spectroscopic information from direct electrical measurements in a device. As the energy level alignment determines the charge injection, it ultimately lies hidden in the current–voltage characteristics of metal/molecular semiconductor/metal stacks. However, by performing direct current ( I )–voltage ( V ) measurements, it is generally difficult to discern between two different contributions to the device resistance: the contact resistance (connected to the interfacial energy barrier) and the resistance of the bulk semiconductor [1] . In this communication we demonstrate precise measurement of the barrier for charge injection in a device in which the contribution of the contact and the bulk resistance are well separated. As a proof of principle, we focus on the interfaces between C 60 and different metals. Several reports show that significant charge transfer takes place at such interfaces, resulting in strong interfacial dipoles and band bending [7] , [8] , [9] , [10] , [11] , [12] , [13] . Here we directly measure the metal/C 60 energy barriers for carrier injection in a vertical device geometry, and study how these barriers determine the in-device electrical resistance. Furthermore, our approach allows the injection of carriers into molecular semiconductors above the energy barrier, thus free from the contact resistance, with interesting implications for spintronics and low-temperature physics. Device scheme and fabrication Our device is based on ballistic electron emission [14] , [15] . This principle has been first applied in microscopy, where a scanning tunnelling microscope tip is used to inject a hot electron current into a thin metal layer deposited on to a semiconductor. An analysis of the current flowing through the semiconductor allows one to obtain information on the interfacial energy barrier. This technique was first applied to the study of the energy barrier at metal/inorganic semiconductor interface [14] , [15] , and only recently it has been applied to metal/molecule systems [16] , [17] . Here we perform ballistic electron emission spectroscopy in a solid-state device by replacing the electron injection from the scanning tunnelling microscope tip with a large-area tunnel barrier. More specifically, our device is composed of an emitter, a base and a collector (as shown in Fig. 1a,b ). The emitter and the base are two metallic electrodes separated by a tunnel junction. The emitter is a 13-nm-thick Al contact that is plasma-oxidized in situ to create a thin AlO x barrier. As a base we employ different metals for the determination of the energy level alignment between them and the adjacent C 60 molecules. A 200-nm-thick C 60 layer serves as a semiconducting collector. A 15-nm-thick Al top electrode is used for the actual electrical contact to C 60 . The energy alignment between the Fermi level of emitter and base is externally controlled with the external bias V EB (see Fig. 1a ), while the energy alignment at the base/collector interface is naturally given by the metal/C 60 energy barrier Δ. 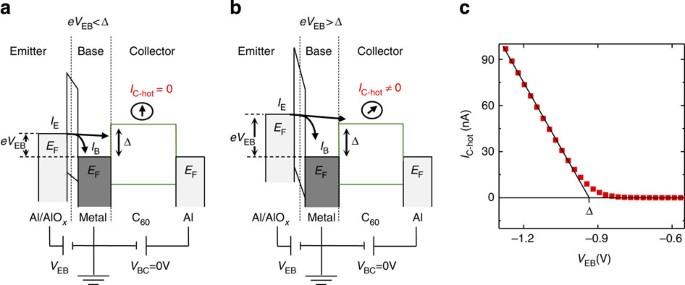Figure 1: Working principle of the device. This working principle is used to measure the energy barrier at metal/C60interfaces. (a,b) Scheme of the energetics of the device.EFrepresents the Fermi energy of the metals. The tunnelling currentIEflows when a biasVEBis applied at the emitter/base terminals. When the biasVEBis lower than the energy barrier Δ at the metal/C60interface,IEflows into the base where it is measured as base currentIB. In this case, no current is measured into the C60(a). When the biasVEBis higher than Δ, part of the tunnelling currentIEflows into the C60and is measured as collector currentIC-hoteven in the absence of an external voltage directly applied across C60(VBC=0) (b). (c) Hot electron currentIC-hotas a function of the applied bias between emitter and baseVEBmeasured at the collector in a device with a 10-nm-thick Cu base at 245 K. The barrier height is Δ=0.95 V, as obtained by interpolating the linear fit of the growth and theI=0 line. Figure 1: Working principle of the device. This working principle is used to measure the energy barrier at metal/C 60 interfaces. ( a , b ) Scheme of the energetics of the device. E F represents the Fermi energy of the metals. The tunnelling current I E flows when a bias V EB is applied at the emitter/base terminals. When the bias V EB is lower than the energy barrier Δ at the metal/C 60 interface, I E flows into the base where it is measured as base current I B . In this case, no current is measured into the C 60 ( a ). When the bias V EB is higher than Δ, part of the tunnelling current I E flows into the C 60 and is measured as collector current I C-hot even in the absence of an external voltage directly applied across C 60 ( V BC =0) ( b ). ( c ) Hot electron current I C-hot as a function of the applied bias between emitter and base V EB measured at the collector in a device with a 10-nm-thick Cu base at 245 K. The barrier height is Δ=0.95 V, as obtained by interpolating the linear fit of the growth and the I =0 line. Full size image When the bias V EB is applied, a current I E is injected from the emitter into the device as electrons tunnel through the AlO x barrier. These injected electrons are regarded as ‘hot’ in the base, because their energy level is well above the Fermi energy level of the metal base. A fraction of these electrons go through the base ballistically with no energy attenuation, provided that the base is sufficiently thin (in a few nanometre range). If the external voltage V EB is lower than the barrier Δ, these ballistic electrons are reflected at the metal/C 60 interface and flow as the base current I B . In this case, all the emitted current I E flows in the base terminal ( I E = I B ) and no collector current is measured ( I C =0, Fig. 1a ). Instead, if V EB >Δ, then some of the hot electrons enter the C 60 layer and diffuse towards the top Al electrode, where they are collected as I C . Since I C generates from the hot electrons in the base, we refer to it as I C-hot . In this case, a part of the emitted current flows into the base and the other part into the collector ( I E = I B + I C-hot , Fig. 1b ). The information about the energy barrier lies in I C-hot ( V EB ), since it is I C-hot =0 for V EB <Δ and I C-hot ≠0 for V EB >Δ (ref. 14 ). A typical measurement of I C-hot versus V EB is shown in Fig. 1c for a device with a 10-nm-thick Cu metal base. Clearly, I C-hot =0 is fulfilled when V EB is below a certain threshold, and then increases roughly linearly [15] . To obtain the barrier height, we employ a simple and visual method as shown in Fig. 1c . We fit the rise of I C-hot above V EB by a linear function over some hundreds of mV and we use the voltage at which the fitting line intercepts I =0 as an approximation of the barrier height. In the case of Fig. 1c , we obtain Δ=0.93 V. We highlight that since C 60 is an n -type semiconductor, we measure the energy barrier between the Fermi level of the metal base and the lowest unoccupied molecular orbital (LUMO) of C 60 , which is the orbital devoted to the charge transport. This also implies that if the base is kept at ground potential ( Fig. 1a,b ), V EB must be negative to inject hot electrons into the base and then into the C 60 layer. Moreover, the current I C-hot is measured without external V BC applied across the C 60 terminals; thus I C-hot can be regarded as a purely diffusive current steaming exclusively from the emitter. Two factors make possible the current flow into the C 60 layer without any externally applied bias. First, the electrons that are injected into the C 60 layer possess a component of the momentum directed perpendicular to the metal/C 60 interface [14] , [15] , with which they diffuse towards the top electrode. Second, inside the C 60 layer there is an internal electric field due to the difference between the work function of the two metals sandwiching the C 60 layer [18] . Since the top Al electrode has the highest work function between all metals of this study (see below), the electric field is always directed to accelerate the electrons towards it. For trap-free inorganic semiconductors, analogous factors—the initial velocity and the acceleration of the electric field present at the metal/semiconductor Schottky barrier—are sufficient for the electrons to diffuse and be collected as current. For this reason, the analysis of the wide majority of the ballistic electron emission experiments based on inorganic semiconductor does not take into account the bulk resistance of the collector [14] , [15] , [19] , [20] , [21] . The electrons allowed to enter into the collector thermalize quickly in the semiconductor [21] , but they are considered free to diffuse into the semiconductor, where they are collected as hot electron current. This assumption is justified in inorganic band-like semiconductors, where the extremely low-defect concentration allows an almost ideal trap-free transport. Indeed, only at very low temperatures (below 10 K) the resistance of inorganic semiconductors was found to play a role in the determination of the magnitude of I C-hot (ref. 22 ). For C 60 , the assumption of trap-free transport is not justified, and we found that the bulk resistance of C 60 has a strong impact on the magnitude of the current I C-hot , as shown in the next section. Electrical characterization When the base material is ferromagnetic, the hot electron current injected in the semiconductor possesses a very high spin polarization [21] , with interesting implications for spintronics [23] . For this reason, throughout this article we mainly focus on the electrical characterization of devices based on a ferromagnetic Ni 80 Fe 20 (NiFe) base. 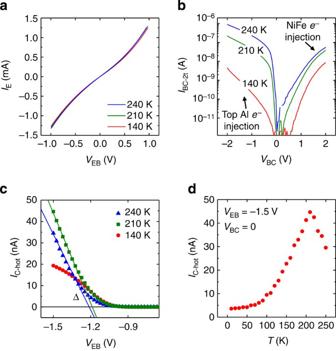Figure 2: Electrical characterization of Al/AlOx/NiFe/C60/Al devices at different temperatures. (a) CurrentIEmeasured at two terminals in the Al/AlOx/NiFe tunnel junction as a function of the applied bias. (b) CurrentIBC-2tmeasured at two terminals in the NiFe/C60/Al stack as a function of the applied bias. Negative and positive polarity correspond to electron injection by the top Al and the bottom NiFe electrodes, respectively. (c) Hot electron currentIC-hotmeasured in the NiFe/C60/Al stack as a function of the applied bias between emitter and base. The barrier height Δ is obtained by interpolating the linear fit of the growth toI=0. (d) Temperature dependence ofIC-hotmeasured atVEB=−1.5 V andVBC=0. Figure 2 shows the typical electrical characterization of a device with a 7-nm-thick NiFe base at three different temperatures. The I–V characteristics of the tunnel junctions are shown in Fig. 2a . The resistance slightly increases when lowering the temperature, as expected for continuous tunnel junctions. Figure 2b shows the I BC-2t – V BC characteristics of NiFe/C 60 /Al stack. In this case the current flowing in the C 60 is driven by a sweep of the voltage V BC directly at the NiFe/C 60 /Al electrodes, so it is a conventional two-terminal measurement comprising the contribution of the contact and the bulk resistance. To avoid confusion with I C-hot , we refer to this as I BC-2t . The temperature evolution of the I BC-2t – V BC traces shows the thermally activated behaviour typical of transport through thick-layer molecular semiconductor [24] . At every temperature, the I BC-2t – V BC characteristics show a diode-like shape. More current flows into the device when electrons are injected by the top Al layer ( V BC <0), while the current injected by the NiFe electrode ( V BC >0) is extremely low below 1 V, suggesting the formation of a high energy barrier at the NiFe/C 60 interface. Figure 2: Electrical characterization of Al/AlO x /NiFe/C 60 /Al devices at different temperatures. ( a ) Current I E measured at two terminals in the Al/AlO x /NiFe tunnel junction as a function of the applied bias. ( b ) Current I BC-2t measured at two terminals in the NiFe/C 60 /Al stack as a function of the applied bias. Negative and positive polarity correspond to electron injection by the top Al and the bottom NiFe electrodes, respectively. ( c ) Hot electron current I C-hot measured in the NiFe/C 60 /Al stack as a function of the applied bias between emitter and base. The barrier height Δ is obtained by interpolating the linear fit of the growth to I =0. ( d ) Temperature dependence of I C-hot measured at V EB =−1.5 V and V BC =0. Full size image Figure 2c shows the I C-hot – V EB characteristics of the device at the same temperatures. Interestingly, the temperature dependence of I C-hot and I BC-2t are very different. In Fig. 2c , we observe that I C-hot at 210 K is higher than that at 240 K, even though I BC-2t of the NiFe/C 60 /Al stack at 210 K is one order of magnitude lower than that at 240 K. This result is explained by the fact that the two-terminal measurement of Fig. 2b is a sum of the contribution of the interface resistance plus the bulk resistance. For a device with a 200-nm-thick molecular layer, the resistance is interface dominated [24] and the current decrease is due to the unfavourable carrier injection. Instead, the current I C-hot flowing in Fig. 2c is not affected by the interface resistance since the electrons are injected above the energy barrier. I C-hot increases because in this temperature range electrons undergo less scattering with phonons in the base, so more electrons are allowed to travel ballistically and reach the collector [20] . The variation of the current I C-hot measured at V EB =−1.5 V in a device with a NiFe base is shown in Fig. 2d . Below 210 K, I C-hot begins to drop as a result of the decreasing mobility of the C 60 film. As in ordinary molecular semiconductors, the mobility of C 60 becomes very low with decreasing temperature [25] , so that the injected electrons cannot diffuse through the whole C 60 film. Instead, they get trapped into shallow traps of the molecular layer, effectively causing the decrease in I C-hot . In this respect, while the ‘onset’ of I C-hot is related to the barrier height, its ‘magnitude’ is related to the electron transport through the bulk C 60 layer. The one-order-of-magnitude decrease in I C-hot between 240 and 10 K is very limited when compared with the variation in I BC-2t , which decreases five orders of magnitude in the same temperature range (the current I BC-2t at 10 K is shown below). Thus, the temperature dependence of the current is a good criterion to confirm the ‘hot electron’ origin of the current I C-hot . An analogous temperature dependence was observed in silicon at much lower temperatures, with the hot electron current decreasing below 10 K [22] . Compared with Si (ref. 22 ), the current in C 60 starts to decrease at much higher temperature. This result is due to the higher numbers of traps of our disordered C 60 layer as compared with Si and it is expected on the basis of the different transport mechanisms in the two materials. In a similar device based on Alq3, the hot electron current could not be measured without externally applied bias since the mobility of Alq3 is too low to allow electrons to diffuse through it even at room temperature [26] . In that case, the electrical characteristics of the device were explained by considering that all the injected electrons would get trapped into the first molecular layer. Effect of the external bias voltage V BC The current I C-hot injected into the C 60 layer at 10 K is shown in Fig. 3a . Following the discussion above, the magnitude of I C-hot is lower at 10 K than at 210 K (compare Figs 2c and 3a ). However, I C-hot can be increased by applying an external bias at the base–collector directed as to accelerate the hot electrons towards the Al collector. As shown in Fig. 3b , when an external bias voltage V BC =3 V is applied the magnitude of I C-hot reaches 300 nA, two orders of magnitude higher than for the case V BC =0. Such an increase can be explained considering that an electric field is capable of removing electrons from shallow traps [27] so that more electrons can contribute to I C-hot . 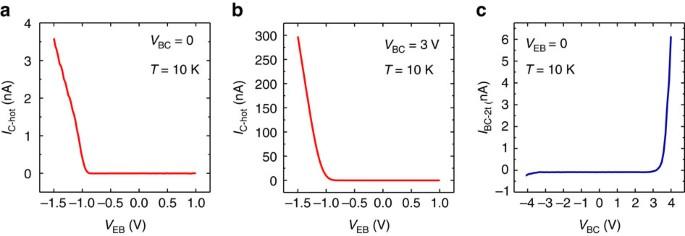Figure 3: Effect of the external bias voltageVBC. CurrentIC-hotas a function of the applied bias between emitter and baseVEBmeasured at 10 K for the same device with different applied bias across the C60film: (a)VBC=0 and (b)VBC=3 V. (c) The two-terminal currentIBC-2tas a function of the biasVBCapplied across the C60at the same temperature. Figure 3: Effect of the external bias voltage V BC. Current I C-hot as a function of the applied bias between emitter and base V EB measured at 10 K for the same device with different applied bias across the C 60 film: ( a ) V BC =0 and ( b ) V BC =3 V. ( c ) The two-terminal current I BC-2t as a function of the bias V BC applied across the C 60 at the same temperature. Full size image We note that at 10 K the two-terminal resistance of C 60 is extremely high, as shown in Fig. 3c . In particular, the current flowing into C 60 driven by the external voltage V BC =3 V is well below 1 nA. Therefore, the current introduced by the direct voltage V BC would not explain the increase in I C-hot . This same experiment could not be performed at temperatures above 200 K, since in that case the current introduced by directly biasing the C 60 film would be higher than the increase in the current I C-hot . We mention that at 10 K it would not be possible to inject a 300-nA current by directly biasing the C 60 layer since one should apply a bias voltage higher than the breakdown voltage of the layer (which was found to be below 6 V). For this reason, we believe that this method could be employed to obtain sizable current intensity flowing in semiconductors at very low temperatures, in a range where the contact resistance usually prevents an efficient carrier injection. Energy barriers at different metal/C 60 interfaces A direct comparison of the measurements of the energy barrier for different base materials (Au, Cu, and NiFe) is shown in Fig. 4 . The work functions of these materials are shown in Fig. 4a compared with the energy levels of C 60 and with the work function of Al, which is used as top electrode in the C 60 collector. Al has the lowest work function, which is quite well matched with the LUMO of C 60 . All the other metals have a work function between the highest occupied molecular orbital (HOMO) and the LUMO. The I BC-2t – V BC traces of all the metal/C 60 /Al present a diode-like I–V characteristic similar to those shown in Fig. 2b for the NiFe base ( Supplementary Fig. 1 ). 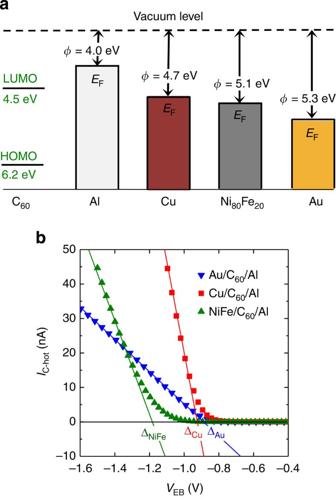Figure 4: Energy barriers at metal C60interfaces. (a) Comparison between the work functionsϕof the different materials used in this study and the molecular levels of C60. The values are taken from ref.1,2. (b) Hot electron currentIC-hotas a function of the applied bias between emitter and baseVEBmeasured in devices with different metal bases: Au, Cu and NiFe. The measurements are carried out at 210 K. The barrier height Δ is obtained by interpolating the linear fit of the growth toI=0. Figure 4: Energy barriers at metal C 60 interfaces. ( a ) Comparison between the work functions ϕ of the different materials used in this study and the molecular levels of C 60 . The values are taken from ref. [1] , [2] . ( b ) Hot electron current I C-hot as a function of the applied bias between emitter and base V EB measured in devices with different metal bases: Au, Cu and NiFe. The measurements are carried out at 210 K. The barrier height Δ is obtained by interpolating the linear fit of the growth to I =0. Full size image In Fig. 4b we show the I C-hot – V EB characteristics measured in the devices with the different metal bases. The thickness of the three bases was chosen to be different to account for the different attenuation length in the different metals. In particular, the energy attenuation length is shorter in ferromagnetic metals, so that we employed a 7-nm-thick NiFe base and 10-nm-thick Cu and Au bases to measure comparable currents. Indeed, the order of magnitude of the currents is the same in the three cases described in Fig. 4 . By contrast, we find that the voltage dependence of the I C-hot turns out to be different. In particular, the slope of the line fitting the experimental data for V EB <Δ is different in the three cases. This is explained as follows. The current reaching the top Al electrode is a fraction of the current flowing into the tunnel junction. Therefore, higher current flowing into the tunnel junction corresponds to higher current getting to the top Al electrode. In the case of Fig. 4b , the resistance of the tunnel junction based on NiFe and Cu are comparable, while the resistance of the Au tunnel junction is one order of magnitude higher ( Supplementary Fig. 2 ), explaining why the increase of I C-hot in the Au device is less steep than the increase in the other two devices. Furthermore, although the C 60 layer was grown always at the same substrate temperature and at the same deposition rate, its transport properties were reproducible only within one order of magnitude, thus introducing some variability on the shape of the I C-hot – V EB trace. Separation of contact and bulk resistance We show now that the device allows distinguishing between the contribution of the interface and of the bulk to the total resistance of C 60 . To do so we measure a device before and after annealing (performed at 10 −6 mbar and 200 °C for 1 h). Again, we focus on a device with a NiFe base. 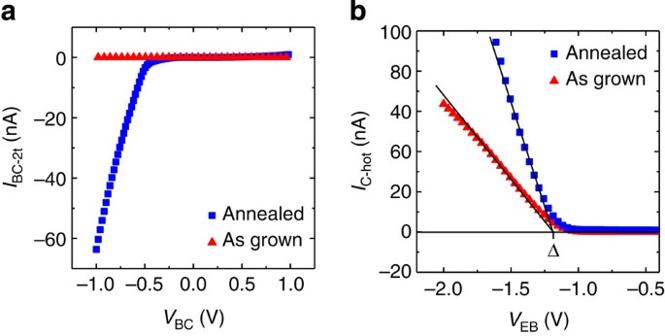Figure 5: Effect of annealing on the device. (a) CurrentIBC-2tmeasured at two terminals in the NiFe/C60/Al stack as a function of the applied biasVBCat 150 K for the same device before and after an annealing process. (b) Hot electron currentIC-hotas a function of the applied bias between emitter and baseVEBmeasured at 150 K for the same device before and after the annealing. In bothI–Vtraces a voltageVBC=1 V is applied during the measurement to increase the measured hot electron current. Figure 5a shows the current I BC-2t as a function of V BC at 150 K before (red) and after (blue) annealing. Clearly, the two-terminal resistance of the NiFe/C 60 /Al stack decreases during the annealing step: before annealing the current I BC-2t at 150 K is extremely low (below the detection limit between −1 V and 1 V), while a significant current amount of flows at the same temperature after the annealing. By considering only the data in Fig. 5a , it would be difficult to understand whether the conductivity change is connected to a modification of the injection barrier or rather to a change in the conductivity of the bulk C 60 . In fact, an interpretation based on a modified barrier was put forward to explain the increase in conductivity measured in a similar structure [28] . In the present case, we could directly measure the barrier height before and after the annealing. Figure 5b shows I C-hot versus V EB before and after the annealing. In both cases, we obtain the barrier height Δ=1.21 V. Thus, the change in the two-point conductivity of the NiFe/C 60 /Al stack is not related to a change in the barrier height, so that it must be due to an improved conductance through the bulk C 60 . Indeed, the annealing improves the ordering of the molecular layer and thus its mobility. Furthermore, we notice that after annealing also the magnitude of the current I C-hot increases. As discussed above, we relate such an increase to the improved conductance of the bulk C 60 . Figure 5: Effect of annealing on the device. ( a ) Current I BC-2t measured at two terminals in the NiFe/C 60 /Al stack as a function of the applied bias V BC at 150 K for the same device before and after an annealing process. ( b ) Hot electron current I C-hot as a function of the applied bias between emitter and base V EB measured at 150 K for the same device before and after the annealing. In both I–V traces a voltage V BC =1 V is applied during the measurement to increase the measured hot electron current. Full size image The energy level alignment is ultimately determined by the electric dipoles that build up at the metal/molecule interfaces [1] , [2] . A ubiquitous contribution to the interface dipole at metal/organic interfaces arises from a rearrangement of the metal electron density on the deposition of the organic layer. At the metal surface, the tail of the electronic density protruding into vacuum is reduced because of the Coulomb repulsion with the molecules. This effect, called push-back or pillow effect, has been reported in different metal/organic surfaces [29] , [30] , [31] and contributes to explain the results of our metal/C 60 interfaces. On the other hand, the energy barrier at the NiFe/C 60 interfaces (Δ=1.2 V) is substantially higher than the energy barriers at Au/C 60 (Δ=0.89 V) and Cu/C 60 (Δ=0.93 V). This result would not be expected on the basis of just the different work functions of the various metals. In particular, Au has the highest work function, so one would expect it to form the highest barrier for electron injection with C 60 . Instead, we find that its barrier is the lowest. This result shows that the work function is not the only important factor for the determination of the interfacial energetics. In fact, in addition to the push-back effect, the amount of transferred charge depends on the material hardness, defined as the derivative of the chemical potential with respect to the number of electrons [32] . The hardness is an indication of the ease of a metal to transfer charge, and it is inversely proportional to the density of states at the Fermi level. Au and Cu have density of state at the Fermi level lower than NiFe, so that they are harder, that is, less prone to donate charge [29] . The interfacial dipoles are expected to be lower than those which build up at the NiFe/C 60 molecule interfaces, nicely explaining the measured differences in energy barriers. Our results are in agreement with spectroscopy data, showing highest hybridization at the C 60 /Ni interface as compared with Au and Cu (refs 10 , 11 ). Furthermore, additional information can be extracted by studying the shape of the increase of I C-hot close to the energy barrier. From Fig. 4b , it is known that the I C-hot – V EB for NiFe is far from the linear fitting we employ to extract the barrier height. This effect can be explained taking into account the density of states of the molecular semiconductor. At the interface, the molecular levels broaden because of the interaction with the metal surface, with a broadening that can be approximated by a Gaussian or a Lorentzian distribution [1] , [2] , [24] . Therefore, the electrons can enter into the semiconductor before reaching the LUMO since they find available states in the tail of the LUMO energy broadening, as schematically shown in Supplementary Fig. 3a . The energy broadening of the LUMO of the C 60 is expected to be quite different in the three cases since it depends on the degree of interaction between the molecules and the metal surface. [1] , [24] Therefore, since NiFe is the metal that interacts the most, the NiFe/C 60 has not only the highest energy barrier, but also the highest energy broadening. In this regard, we believe that the shape of the current increase at the cut-off returns information on the shape of the density of states in the molecular film. In Supplementary Note 1 we develop a detailed model that takes into account the density of states of the molecular semiconductor to fit the data of Fig. 4 . By employing such model, we can closely reproduce the shape of the curves as shown in Supplementary Fig. 3 . Finally, we discuss how this device scheme can be further extended to other experimental situations. From a technical point of view, the device production and measurement does not present particular complications and can be readily reproduced. Basically, the structure of our device is nothing but a metal/semiconductor/metal stack grown on an Al/AlO x contact, which serves as electron injector. The Al/AlO x contact is in turn easy to produce since Al is widely used in organic electronics and the AlO x thin barrier can be obtained by exposing the Al layer to oxygen plasma, which is available in the vast majority of physical/chemical laboratories. To obtain the information about the energy barrier, one needs to adopt a conventional three-terminal measurement in which one bias voltage is kept fixed and another one is swept—analogous to the basic measurements of any kind of transistors. Furthermore, in Supplementary Figs 4 and 5 we show the results of devices produced ex situ . If gold is employed as the base material, the barrier height can be measured even in a device that was exposed to air for 20 min before the C 60 deposition (see also Supplementary Note 2 ). Without the requirement of in situ deposition, a large variety of metal/semiconductor interfaces can be studied with the present method, including small molecules and polymers deposited via wet methods and solution-processable perovskites. Even lateral geometries for the devices are conceivable and have been demonstrated for inorganic semiconductors [33] , paving the way to the study of two-dimensional layered systems. Only semiconductors with very low mobility are not suitable in devices similar to those presented since the hot electron current would not diffuse through them. However, the materials of interest for applications in electronics possess relatively high mobility, so even this requirement does not represent a limitation. Furthermore, whereas in this communication we demonstrate only the measurement of the energy barriers for electrons, information on the injection barrier for holes can also be obtained [34] , extending even further the range of applicability of this method. In conclusion, we have shown that the energy alignment at metal/molecule interfaces can be measured in a chip by the fabrication of a simple three-terminal device. As a proof of principle, we measured the energy barriers at the interfaces between C 60 and different metals. Furthermore, such a device can be used to inject carriers in the organic layer overcoming the contact resistance. This property allows the injection of a highly spin-polarized current into a molecular layer, which would be a breakthrough in the field of spintronics, or studying its conduction properties at very low temperatures, in a range where the contact resistance usually prevents any carrier injection. We anticipate that this scheme for charge injection free from the contact resistance is not limited to bulk semiconductors but can be extended in principle to any semiconductor, including solution-processable and two-dimensional layered semiconductors. Device preparation All the devices described in this communication were fabricated in situ in a UHV dual chamber evaporator (base pressure <10 −9 mbar) with a shadow mask system. In the Supplementary Information , we show that even a device produced ex situ has the same electrical behaviour. The sample size is 10 × 10 mm 2 , and six devices were produced in every sample. Typical device area is 300 × 300 μm 2 . The measurements were very much reproducible between devices produced in the same evaporation. Metals were e-beam evaporated in one of the chambers at a rate of 0.1 nm s −1 , while C 60 was evaporated in the second one from a Knudsen cell at a rate of 2 nm min −1 . Metals were 99.95% purity (Lesker), while C 60 was of triple-sublimed quality (99.9%) (Sigma Aldrich) and used without further purification. Electrical characterization Electrical characterization was performed under vacuum in a variable-temperature probe station (Lakeshore) after the samples had been exposed to air for ~1 min. A Keithley 4200 semiconductor analyser system was used to record I – V . How to cite this article: Gobbi, M. et al. Determination of energy level alignment at metal/molecule interfaces by in-device electrical spectroscopy. Nat. Commun. 5:4161 doi: 10.1038/ncomms5161 (2014).